A monolithically integrated plasmonic infrared quantum dot camera In the past few years, there has been increasing interest in surface plasmon-polaritons, as a result of the strong near-field enhancement of the electric fields at a metal–dielectric interface. Here we show the first demonstration of a monolithically integrated plasmonic focal plane array (FPA) in the mid-infrared region, using a metal with a two-dimensional hole array on top of an intersubband quantum-dots-in-a-well (DWELL) heterostructure FPA coupled to a read-out integrated circuit. Excellent infrared imagery was obtained with over a 160% increase in the ratio of the signal voltage ( V s ) to the noise voltage ( V n ) of the DWELL camera at the resonant wavelength of λ =6.1 μm. This demonstration paves the way for the development of a new generation of pixel-level spectropolarimetric imagers, which will enable bio-inspired (for example, colour vision) infrared sensors with enhanced detectivity ( D *) or higher operating temperatures. Infrared imagers operating in the 3–12 μm range are useful for a variety of applications ranging from night vision to non-invasive medical diagnostics [1] . The past decade has witnessed dramatic advances in infrared imaging technology with the introduction of new materials such as quantum dots [2] and superlattices [3] , which are posing a challenge to the 50-year incumbent technologies (HgCdTe and InSb). Focal plane array (FPA) technology has progressed from a first generation of single pixel and linear arrays (1960–70s), through a second generation of small format (128×128/256×256) 2D arrays (1980–90s) to a third generation of large format (4×4 K), dual band and higher operating temperature imagers [4] . However, to date all of the pixels in an infrared camera are as close to identical as possible, thus presenting only a 'black and white' version of a scene. In contrast, imagers found in nature such as the human eye encode information such as colour, dynamic range and polarization at the pixel level. The quantum dots were grown using solid source molecular beam epitaxy (MBE) using a Stranski–Krastonow growth mode, in which strain driven dynamics drive the formation of the dots similar to the processes that lead to the self-assembly of oil droplets on a water surface [5] . In particular, the dots-in-a-well (DWELL) detector architecture pioneered at the University of New Mexico was used as a prototype in these studies [6] , [7] . The DWELL architecture is a hybrid structure in which InAs quantum dots are placed in an InGaAs quantum well. The DWELLs combine the good control over the operating wavelength of quantum-well infrared photodetectors with the low dark current and normal incidence operation of quantum dot infrared photodetectors. In the meanwhile, there has been increasing interest in the strongly enhanced electric fields in the local vicinity of a resonant coupling surface plasmon-polariton (SPP) structure such as a metal film perforated with a one-dimensional slit or two-dimensional (2D) hole array [8] . Various optoelectronic devices, such as lasers, detectors, filters and solar cells, are expected to benefit from this enhancement, which allows spectropolarimetric control over emission and detection processes [9] , [10] . Various nanostructure architectures for enhanced-field couplers have been explored in the literature, including bull's eye, bow-tie, C-aperture and periodic inductive and capacitive arrays [11] , [12] , [13] , fabricated by a wide variety of lithography techniques such as e-beam lithography, ion-beam lithography, nano-imprinting and interferometric lithography (IL) [14] , [15] , [16] , [17] . For this study, we choose a 2D periodic hole array, which is easy to fabricate using IL [17] . These surface plasmon (SP) structures could be readily adapted into conventional FPA processing flows, as the feature sizes (1- to 3-μm) that are needed for infrared imagers are easily defined using standard optical lithography. In this paper, we demonstrate the first monolithically integrated plasmonic camera using near field spectrally resonant coupling of the SPPs with infrared absorption in the quantum dots as an important step towards this broader, biomimetic vision of infrared imaging. Moreover, the plasmonics approach is detector agnostic and can be introduced into a standard imaging camera fabrication process using a single photolithography step. 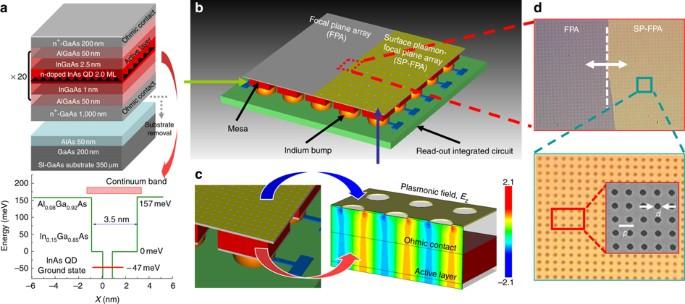Figure 1: Schematic of the plasmonic dots-in-a-well (DWELL) focal plane array. (a) Heterostructure schematic and band diagram of the DWELL absorber. (b)Schematic view of the surface plasmon (SP) structure defined on one half of the DWELL FPA after hybridization with a read-out integrated circuit (ROIC) and subsequent substrate removal. (c) Zoomed-in image showing the FPA bonded to the ROIC along with the SP electric field (Ez) profile. (d) Visible images of the two halves of the FPA clearly showing the non-plasmonic and plasmonic sections. The orthogonal pitches of the two-dimensional grating are both fixed at 1.79 μm (p). The metal thickness is about 50 nm. The circular aperture size (d) is fixed at 0.5p. Design and fabrication of plasmonic infrared DWELL FPA Figure 1 shows a schematic diagram of the monolithically integrated quantum dot FPA with zoomed-in images of the heterostructure and a band diagram of the absorber, details of the SP structure and the simulated z -component of SP electric field. The absorber consists of 20 stacks of a InAs/In 0.15 Ga 0.85 As DWELL structure sandwiched between two n-GaAs contact layers of 200 nm (top) and 1,000 nm (bottom), respectively, and separated from the substrate by a 50 nm AlAs etch-stop barrier. After the epitaxial growth (details in Methods), the wafer was processed into a 320×256 (¼ VGA) FPA with a 30 μm pixel pitch using standard optical lithography, inductively coupled plasma etching, plasma-enhanced chemical vapour deposition of SiN x , contact metal and under-bump metal deposition. Indium bumps were deposited, the FPA was hybridized to an Indigo 9705 read-out integrated circuit (ROIC), and the substrate was removed using a series of mechanical polishing and dry etching steps ending at the 50 nm AlAs etch-stop layer. The detailed processing sequence is included in the Methods. Figure 1: Schematic of the plasmonic dots-in-a-well (DWELL) focal plane array. ( a ) Heterostructure schematic and band diagram of the DWELL absorber. ( b )Schematic view of the surface plasmon (SP) structure defined on one half of the DWELL FPA after hybridization with a read-out integrated circuit (ROIC) and subsequent substrate removal. ( c ) Zoomed-in image showing the FPA bonded to the ROIC along with the SP electric field ( E z ) profile. ( d ) Visible images of the two halves of the FPA clearly showing the non-plasmonic and plasmonic sections. The orthogonal pitches of the two-dimensional grating are both fixed at 1.79 μm ( p ). The metal thickness is about 50 nm. The circular aperture size ( d ) is fixed at 0.5 p . Full size image Following the substrate removal, a 2D periodic SP inductive (hole) array was fabricated using IL, e-beam metal evaporation and lift-off processing. Half of the FPA was protected with a thick polymer layer during this fabrication that was later removed (see Methods for more details). A 1,000 nm bottom contact layer separated the DWELL layer from the SP array, which slightly impacts the overlap between the SPP field and the absorption region. To determine the optimized SP structure to integrate with the FPA, a series of square symmetry 2D Ti/Au SP hole arrays were fabricated on a 1,000 nm epitaxially grown n-GaAs (2×18 cm −3 ) layers with pitches ranging from 1.79 to 2.33 μm. A 2D square array of circular apertures was formed with a nominal ratio of diameter d to lattice spacing p , d / p ∼ 0.5. The normal incidence transmission was measured using a Fourier transform infrared (FTIR) spectrometer and was normalized to the transmission through a bare substrate. Experimental and simulated SP resonances For normal incidence geometry, the SP resonance wavelengths are given by where i and j are integer indices indicating the order of the coupling, p is the pitch of the SP structure, ɛ k is the complex permittivity ( ɛ k = ɛ k ′+i ɛ k ″, where k =d (dielectric) or m (metal)) [10] , [13] , [18] . The electromagnetic field profile of the SP structure was modelled using both a finite integration technique (CST Microwave Studio, CST Studio Suite ( www.cst.com )) and a rigorous coupled-wave analysis [19] , [20] . The refractive index of the material ( n eff ) was taken to be the effective index of the first order resonance of SP modes ( ∼ λ 1,0 / p ) and the Drude model for the gold dielectric function at frequencies of interest is described by a plasma frequency ω p =9.02 eV and a scattering frequency ω c =0.027 eV (refs 21 , 22 ). As expected, the resonance wavelengths linearly increased with the pitch. 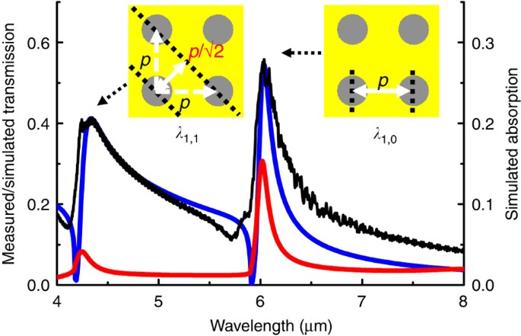Figure 2: Transmission spectrum of plasmonic structures. Measured transmission (black line) and simulated transmission (blue line)/absorption (red line) obtained from a 1,000 nm n-GaAs layer obtained using Fourier transform infrared (FTIR) spectrometer and rigorous coupled-wave analysis simulation showing good agreement between the experimental measurement and the theoretical calculation. The pitch corresponding to the two resonances are shown in the inset to the figure. A pitch of 1.79 μm was used in the fabrication of the SP on the DWELL FPA. The experimentally measured resonances demonstrate very good agreement with the theoretically simulated transmission spectra, also shown in Figure 2 . A pitch of 1.79 μm was chosen for the SP array for the FPA integration corresponding to a (1,0) resonance of ∼ 6.1 μm and a (1,1) resonance of ∼ 4.3 μm. Figure 2: Transmission spectrum of plasmonic structures. Measured transmission (black line) and simulated transmission (blue line)/absorption (red line) obtained from a 1,000 nm n-GaAs layer obtained using Fourier transform infrared (FTIR) spectrometer and rigorous coupled-wave analysis simulation showing good agreement between the experimental measurement and the theoretical calculation. The pitch corresponding to the two resonances are shown in the inset to the figure. A pitch of 1.79 μm was used in the fabrication of the SP on the DWELL FPA. 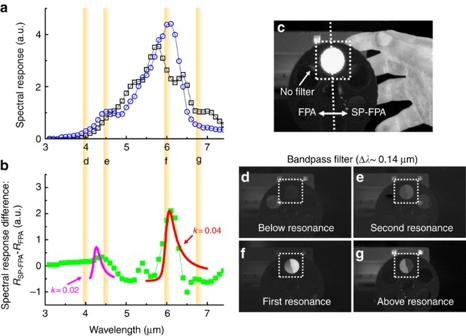Figure 3: Spectrally resonant enhancement in plasmonic DWELL camera. (a) Spectral response of the two halves of the plasmonic FPA using a monochromator system. Blue, spectral response of SP-FPA; black, spectral response of FPA. (b) Difference plot showing the experimentally observed peaks. The theoretically modelled (1,0) and (1,1) SP resonances are also shown usingk=0.04 andk=0.02, respectively (kis the imaginary part of the semiconductor dielectric function dominated by the quantum dot infrared photodetector absorption). Green, difference of spectral response between SP-FPA and FPA; red (magenta), theoretically modelled first (second) order SP resonances usingk=0.04 (0.02). (c) Representative image of the blackbody seen through the open slot (no filter) in the filter wheel assembly. Note the clear image of the human hand clearly showing temperature differences of <50 mK. Infrared image of the blackbody (d) below the (1,1) resonance atλ=3.99 μm, (e) near the (1,1) resonance,λ=4.54 μm, (f) close to the (1,0) resonance,λ=5.95 μm and (g) beyond the (1,0) resonance,λ=6.83 μm. It is clear that at the (1,0) and (1,1) resonances, the response of the SP-FPA is brighter than that of the non-SP-FPA, whereas the effect is reversed off resonance. This is in very good agreement with the independent spectral response measurements shown ina. Full size image Characterization of plasmonic infrared DWELL FPA The spectral responses of the two FPA sections (with and without the plasmonic coupler) were measured using a monochromator ( f /4) and are shown in Figure 3a . Resonance enhancement of the response was observed at λ ∼ 4.3 μm and λ ∼ 6.1 μm and is clearly visible in the difference plot shown in Figure 3b . The simulated absorption (arbitrary units) provides a good quantitative agreement for both resonances in terms of wavelength, linewidth and relative strengths. The indicated absorption (corresponding to n +i k ) is due to the quantum dot infrared photodetectors material; was adjusted to fit to the measurement; and provides a qualitative estimate of the propagation length along the pixel. A k =0.04 corresponds to a SP absorption length of ∼ 12 μm, less than the pixel linear dimension and much less than the SP '1/ e ' length of ∼ 0.2 mm from the metal losses alone. Figure 3c shows the image of a blackbody using f /2.3 optics seen through an open slot (no filter) of a filter wheel assembly. The excellent image quality is reflected in the infrared image of the hand, with temperature differences of 50 mK being captured by the plasmonic imager. A series of visual images of the resonant enhancement was obtained using narrow band filters (Δ λ =140 nm) placed in front of the blackbody. Four different cases are shown in Figure 3d–g . Below the (1,1) resonance ( λ =3.99 μm), there is only a very small difference between the SP and the non-SP halves of the FPA. In the vicinity of the (1,1) resonance ( λ =4.54 μm), the SP-half of the FPA appears slightly brighter than the non-SP half of the FPA. Close to the (1,0) resonance ( λ =5.95 μm), there is a clear enhancement of the SP-half of the FPA. Past the (1,0) resonance ( λ =6.83 μm), the non-SP portion of the FPA appears brighter. These observations correlate very well with the measured spectral responses as shown in Figure 3b . Figure 3: Spectrally resonant enhancement in plasmonic DWELL camera. ( a ) Spectral response of the two halves of the plasmonic FPA using a monochromator system. Blue, spectral response of SP-FPA; black, spectral response of FPA. ( b ) Difference plot showing the experimentally observed peaks. The theoretically modelled (1,0) and (1,1) SP resonances are also shown using k =0.04 and k =0.02, respectively ( k is the imaginary part of the semiconductor dielectric function dominated by the quantum dot infrared photodetector absorption). Green, difference of spectral response between SP-FPA and FPA; red (magenta), theoretically modelled first (second) order SP resonances using k =0.04 (0.02). ( c ) Representative image of the blackbody seen through the open slot (no filter) in the filter wheel assembly. Note the clear image of the human hand clearly showing temperature differences of <50 mK. Infrared image of the blackbody ( d ) below the (1,1) resonance at λ =3.99 μm, ( e ) near the (1,1) resonance, λ =4.54 μm, ( f ) close to the (1,0) resonance, λ =5.95 μm and ( g ) beyond the (1,0) resonance, λ =6.83 μm. It is clear that at the (1,0) and (1,1) resonances, the response of the SP-FPA is brighter than that of the non-SP-FPA, whereas the effect is reversed off resonance. This is in very good agreement with the independent spectral response measurements shown in a . Full size image Radiometric characterization of the plasmonic FPA was undertaken using a calibrated blackbody source along with the narrow bandpass filters. 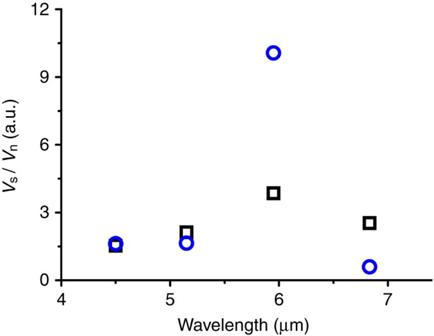Figure 4: Radiometric characterization of plasmonic FPA. Ratio of measured signal voltage (Vs) to noise voltage (Vn) of the detector off and on the SP resonance. The enhancement ofVs/Vnat the first order resonance is increased by over 160%, for this unoptimized structure. Blue,Vs/Vnof SP-FPA; black,Vs/Vnof FPA. Figure 4 depicts the ratio of V s to V n in which the enhancement is more than 160%. The difference in the enhancement factor between the measurements done with the monochromator ( Fig. 3 ) and the narrow band pass filters ( Fig. 4 ) could be due to the sensitivity of the measurements to the angle of incidence as the radiometric measurements were at a smaller f/# (closer to normal incidence) than the spectral measurements. The single pixel results indicate that further improvements are likely with more optimized coupling structures; normal incidence enhancements of ×30 have been reported [23] . This will result in a decrease in the minimum temperature difference that can be recorded by an infrared imager or to an increase in the operating temperature of the camera for the same signal to noise. This is especially important for quantum dot (QD)-based detectors, which have lower dark currents compared with quantum-well infrared photodetectors and type II strained-layer superlattices, but suffer from poor quantum efficiency. Alternatively, this allows a reduction in the active volume of superlattice detectors to reduce the dark current while retaining a high quantum efficiency. The demonstration of this performance enhancement in a full FPA format, validating the single pixel results and demonstrating the applicability to small (24 μm pixels), the absence of obvious crosstalk effects, and the applicability to realistic angular acceptances is an important step towards the integration of plasmonic structures into next generation infrared FPAs. Figure 4: Radiometric characterization of plasmonic FPA. Ratio of measured signal voltage ( V s ) to noise voltage ( V n ) of the detector off and on the SP resonance. The enhancement of V s / V n at the first order resonance is increased by over 160%, for this unoptimized structure. Blue, V s / V n of SP-FPA; black, V s / V n of FPA. Full size image The present work opens up a huge optimization parameter space. Different SP structures, such as bull's eye, C-aperture and bow-tie aperture, need to be investigated and the resonant enhancement as a function of the field of view needs to be studied. Moreover, these structures can be integrated into the front side processing of the FPA, under the indium bumps, thereby enabling the fabrication of these structures at the wafer level (as opposed to the die level processing reported here). Single pixel results indicate the viability of this approach [24] . The biggest impact of this work will be realized when plasmonic structures with different spectral, polarimetric and dynamic range structures are integrated into each pixel, thereby adding new functionality to an infrared FPA. We can combine this with efficient on-chip compressive sensing algorithms to reduce the data volume while increasing the information from the sensor. This approach of combining a powerful multimodal sensor with ultra-efficient data compression techniques has been perfected by nature. The human eye for instance has a retina with over 150 million photoreceptors. But the amount of data that is fed into the optic nerve, which only has 1 million nerve endings, is compressed by at least 2 orders of magnitude. Scientists now believe that the retina only sends 10–12 compressed images to the brain for the reconstruction of a rich visual image with this sparse data [25] . Thus, the human eye has the ability to sense a huge amount of multimodal data but also has the intelligence to output only a small fraction for analysis. We believe that this work enables us to get one step closer to our vision of realizing a bio-inspired spectropolarimetric sensor. Epitaxial growth of quantum DWELL infrared photodetector The detector structure was grown on a 2-inch semi-insulating GaAs substrate with a solid source MBE machine equipped with an As 2 cracker source. A GaAs buffer layer was grown to smooth the surface before the device layer growth. A 50-nm AlAs etch stop layer was then grown, followed by 1,000 nm n-doped GaAs bottom contact layer (Si doped, n =2×10 18 cm −3 ). The active layer consists of 20 periods of InAs quantum dots embedded in 3.5-nm thick In 0.15 Ga 0.85 As-Al 0.08 Ga 0.92 As quantum wells, each separated by 50-nm Al 0.08 Ga 0.92 As barriers. InAs quantum dots were deposited at 0.053 monolayer/s growth rate at 470 °C substrate temperature. The substrate temperature was ramped to 590 °C for the growth of Al 0.08 Ga 0.92 As barrier layers and GaAs contact layers. The growth rates, substrate temperatures and the flux ratios were previously optimized [26] for maximizing the photoluminescence intensity from the quantum dots. Quantum dots were n-doped with Si with approximately two electrons per dot, for optimizing [27] the detector performance. The thickness and compositions of In 0.15 Ga 0.85 As and Al 0.08 Ga 0.92 As layers were selected to achieve broadband detector response with bound to continuum type of transitions. The single pixel characterization of these detectors has been previously published [28] . The room temperature photoluminescence data obtained with He-Ne laser excitation are plotted in Supplementary Figure S1 . Fabrication of the plasmonic hybrid FPA chip The processing scheme of the plasmonic FPA chip consists of a dry etch to form the mesa, surface passivation, ohmic metal evaporation, under bump metallization, indium deposition and indium reflow processes as shown in Supplementary Figure S2a–g . A 320×256 array mesa with a single pixel area of 24×24 μm 2 and 30 μm pitch was formed using standard optical lithography, inductively coupled plasma etching by BCl 3 gas. A 200-nm thick Si 3 N 4 was deposited for surface passivation using plasma-enhanced chemical vapour deposition. After making a through the Si 3 N 4 , the ohmic contact metals of Ge(280 Å)/Au(540 Å)/Ni(200 Å)/Au(3,000 Å) were deposited by e-beam evaporation, and a rapid thermal anneal (RTA) was performed. This was followed by under bump metallization of Ti(300 Å)/Ni(1,500 Å)/Au(500 Å) and indium deposition of 3 μm thickness. After this, the deposited indium was reflowed to form indium bumps with a height over 8 μm using flux (TAC Flux 019: Indium). The fabricated FPA devices were subsequently hybridized with an Indigo 9705 silicon ROIC chip through a standard flip-chip bonding process at 170 °C using a flip chip bonder (FC150: SUSS MicroTec). To provide mechanical support between FPA and ROIC, underfill epoxy was injected between the FPA and ROIC with the aid of the capillary force as shown in Supplementary Figure S3h,i . The entire substrate was removed and a plasmonic structure was defined on ½ of the back-side of the epilayer, that is, on the top-side of hybrid FPA chip ( Supplementary Fig. S2j ). The GaAs substrate of 350 μm thickness was removed using a series of mechanical polishing and selective dry etching using BCl 3 /SF 6 gases to a 50 nm AlAs etch stop layer. Once the substrate was removed up to the etch stop layer, the AlAs etch stop layer was removed with a hydrofluoric acid solution. Following substrate removal, half of the FPA was covered with a sacrificial photoresist (PR) layer and a periodic 2D square hole SP array was fabricated using IL to define the 2D square symmetry hole array along with e-beam metal evaporation and lift-off processing (details in Supplementary Information : SP structure fabricated by interferometric lithography) as shown in Supplementary Figure S2k . The SP metal consisting of Ti(5 nm)/Au(45 nm) was evaporated ( Supplementary Fig. S2l ). Supplementary Figure S3 shows the schematic, visible and SEM images of various stages of the fabrication processes. The fabricated plasmonic FPA is shown in Supplementary Figure S3c . Surface plasmon structure fabricated by interferometric lithography The processing steps to fabricate the SP structure with circular apertures are as follows. (I) A positive-tone PR (SPR 505A: Shipley) was spin-deposited at 4000 r.p.m. for 30 s and oven-baked at 95 °C for 3 min. (II) IL using a 355-nm 3rd YAG:Nd 3+ laser source was carried out to produce a periodic circular hole pattern in the PR layer with two successive orthogonal one-dimensional exposures with power 50 mJ and same doses to provide a symmetrical aperture shape; a 1 min post-bake at 110 °C was used; the exposed and post-baked sample was developed (MF-702: Shipley) for 1 min and rinsed with deionized water as shown in Supplementary Figure S4a . (III) After the PR pattern was defined, consecutive e-beam evaporations were used to deposit a 5-nm thick layer of titanium (Ti) as an adhesion layer on the developed sample and a 45-nm thick layer of gold (Au) at a pressure of the order of 10 −7 Torr during deposition and ∼ 0.02 nm s −1 , followed by a lift-off processing with a acetone to remove the PR layer as shown in Supplementary Figure S4b [29] . FTIR transmission measurement and simulation based on a finite integration technique To find the optimized SP structure for integration with the FPA, SP structures with various pitches (that is, p =1.79, 1.89, 2.0, 2.08 and 2.33 μm) were fabricated on substrate consisting of a 1 μm thick n-type GaAs layer (2×10 18 cm −3 ) grown on a semi-insulating GaAs wafer by MBE. A 2D square array of circular holes was formed with a ∼ 1:1 line/space ratio). IL was used to fabricate large area (1.5×1.5 cm 2 ), uniform samples and making sample characterization convenient [30] as described above. The transmission was recorded with a Nicolet FTIR spectrometer with a KBr beam splitter and a DTGS-KBr detector. The linear transmission spectra were measured at a normal incidence and normalized to the transmission through a bare substrate as shown in Supplementary Figure S5a . In case of symmetric SP structure with circular apertures, an unpolarized FTIR beam was used to measure the transmission. The wavelength of the first order SP resonance is given by This result can be simplified to and as shown in Supplementary Figure S5b . In addition, a finite integration technique (CST Microwave Studio) was used to obtain the electromagnetic field distribution resulting from the SP structure as shown in Supplementary Figure S5c . Both perfect electric conductor and perfect magnetic conductor boundary conditions were used to stimulate transverse electromagnetic plane wave propagating between unit cells. Characterization of plasmonic infrared DWELL camera The hybrid FPA was mounted in a pour-fill Dewar and cooled down to liquid nitrogen temperature at 77 K. The FPA was connected to a commercial CamIRa FPA demonstration system manufactured by SE-IR Corporation using f /2.3 optics. This system controls the clock, the synchronizations (frame and line) and the FPA bias voltages and interfaces to the hybridized ROIC. The ROIC reads the pixels (the image data) and sends the outputs serially to a computer port. The computer interfaced to this system performs the data processing and storage. With this setup, the spectral responses of FPA and SP-FPA were measured at the bias of 0.3 V as a monochromatic light provided by a PIActon Spectra Pro 2150i monochromator ( f /4 optics) was tuned from 3 to 8 μm in a step of 0.1 μm. The entire test setup for FPA spectral measurement is illustrated in Supplementary Figure S6 . At each wavelength, the FPA output was stored and averaged over 30 frames. Based on the measured spectra of FPA and SP-FPA, the visual demonstration was conducted by placing a filter wheel in front of an OMEGA blackbody source at 150 °C. A filter wheel consists of four narrowband optical filters with centre wavelengths at 3.99, 4.54, 5.95 and 6.83 μm and a bandwidth (Δ λ ) of 140 nm. A total of five different images were captured and displayed for cases of no filter and four different filters to visually inspect the effect of SP-FPA as compared with FPA. For a radiometric characterization of SP-FPA, the device sensitivity [31] , [32] , [33] was considered and obtained by taking the ratio of the signal voltage ( V s ) to the noise voltage ( V n ). The V s was measured by the FPA camera system seen the calibrated blackbody source through the narrowband filter with Δ λ ∼ 140 nm as shown in Supplementary Figure S7 . The measurement was performed for four different wavelengths (4.54, 5.15, 5.95 and 6.83 μm). For each measurement, the corresponding temporal noise voltage V n was obtained by computing the standard deviation of the V s over 30 frames. How to cite this article: Lee, S. J. et al . A monolithically integrated plasmonic infrared quantum dot camera. Nat. Commun. 2:286 doi: 10.1038/ncomms1283 (2011).